Remodelling of the active presequence translocase drives motor-dependent mitochondrial protein translocation Proteins with N-terminal targeting signals are transported across the inner mitochondrial membrane by the presequence translocase. To drive precursor translocation, the Hsp70-import motor associates with the protein-conducting channel of the TIM23 complex. It is unknown how the ATPase cycle of Hsp70 is regulated in the context of a translocating polypeptide chain. Here we establish an assay to monitor protein dynamics in the precursor-occupied presequence translocase and find that regulatory subunits of the import motor, such as the ATPase-stimulating J-protein Pam18, are recruited into the translocation intermediate. The presence of all Hsp70 co-chaperones at the import channel is not sufficient to promote matrix protein import, instead a recharging of the active translocase with Pam18 is required for motor activity. Thus, a replenishment cycle of co-chaperones at the TIM23 complex is an integral part of Hsp70’s ATPase cycle at the channel exit site and essential to maintain motor-driven mitochondrial protein import. Post-translational protein transport across cellular membranes is driven by nucleotide-hydrolysing chaperones that transiently associate with their corresponding protein-conducting channel to bind the unfolded translocating polypeptide chain. For the generation of directional precursor movement, the chaperone’s nucleotide-cycle has to be coupled to the translocase’s activity [1] , [2] , [3] , [4] , [5] . In mitochondria, matrix translocation of polypeptides depends on the ATP-powered mitochondrial Hsp70 (mtHsp70), the catalytic constituent of the presequence translocase-associated motor (PAM), at the trans side of the protein-conducting channel [5] , [6] , [7] , [8] . During precursor transport, a translocation intermediate is established in which the motor-associated, unfolded precursor simultaneously spans the TOM and TIM23 complexes thereby generating a mitochondrial contact site. mtHsp70 exists in a soluble pool mediating matrix protein folding and a TIM23-associated pool generating precursor velocity over the inner membrane. For both activities, the soluble co-chaperone Mge1 stimulates ADP/ATP exchange [9] , [10] . Although matrix co-chaperones act as J-proteins stimulating the ATPase activity of mtHsp70 during protein folding, a TIM23 complex-associated membrane integral J-protein (Pam18) is import specific [11] , [12] , [13] , [14] , [15] . At the resting translocase, Pam18 forms a complex with the J-like Pam16. This association maintains Pam18 in an inactive state [12] , [16] , [17] . The translocase-associated Tim44 is thought to position mtHsp70 at the trans side of the Tim23 channel ( Fig. 1a ) [12] , [18] , [19] . Thus, four essential co-chaperones are required at the translocase to regulate mtHsp70 function during protein import [20] , [21] . 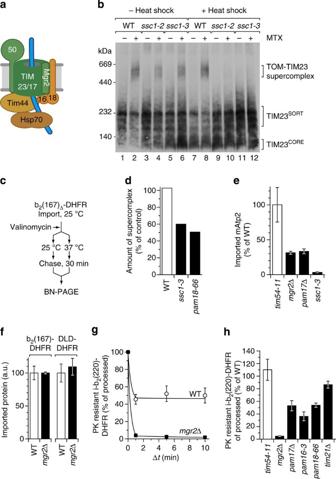Figure 1: Preserving a TOM/TIM23-spanning translocation intermediate requires import motor activity. (a) Model of TIM23 complex with associated import motor and a substrate (blue). (b) Isolated mitochondria were subjected to heat shock before import of purified b2(167)Δ-DHFR in the presence or absence of methotrexate (MTX). Samples were analysed by BN-PAGE and α-Tim23 western blotting. (c) Experimental scheme to assess maintenance of TOM/TIM23-spanning translocation intermediate in temperature-sensitive mutants. (d) Quantification of TOM/TIM23 translocation intermediates after motor inactivation. Amount of supercomplex retained after 37 °C chase (100%; supercomplex retained during 25 °C chase). (e) Import of [35S]Atp2 into isolated WT and mutant mitochondria (mean±s.e.m.,n=3). (f) Import of sorted precursors into isolated WT andmgr2Δ mitochondria (mean±s.e.m.,n=3). (g) Inward driving activity on arrested [35S]b2(220)-DHFR. After import in the presence of MTX, Δψ was dissipated before a second incubation at 25 °C for the indicated time. Samples were PK treated and the amount of the intermediate quantified (100%; processed intermediate without protease treatment, mean±s.e.m.,n=3). (h) Inward driving activity assayed at 5 min chase time in indicated mutant and respective WT mitochondria as described ing(mean±s.e.m.,n≥3). Figure 1: Preserving a TOM/TIM23-spanning translocation intermediate requires import motor activity. ( a ) Model of TIM23 complex with associated import motor and a substrate (blue). ( b ) Isolated mitochondria were subjected to heat shock before import of purified b 2 (167) Δ -DHFR in the presence or absence of methotrexate (MTX). Samples were analysed by BN-PAGE and α-Tim23 western blotting. ( c ) Experimental scheme to assess maintenance of TOM/TIM23-spanning translocation intermediate in temperature-sensitive mutants. ( d ) Quantification of TOM/TIM23 translocation intermediates after motor inactivation. Amount of supercomplex retained after 37 °C chase (100%; supercomplex retained during 25 °C chase). ( e ) Import of [ 35 S]Atp2 into isolated WT and mutant mitochondria (mean±s.e.m., n =3). ( f ) Import of sorted precursors into isolated WT and mgr2 Δ mitochondria (mean±s.e.m., n =3). ( g ) Inward driving activity on arrested [ 35 S]b 2 (220)-DHFR. After import in the presence of MTX, Δψ was dissipated before a second incubation at 25 °C for the indicated time. Samples were PK treated and the amount of the intermediate quantified (100%; processed intermediate without protease treatment, mean±s.e.m., n =3). ( h ) Inward driving activity assayed at 5 min chase time in indicated mutant and respective WT mitochondria as described in g (mean±s.e.m., n ≥3). Full size image Here we establish an experimental approach to analyse protein dynamics of an active translocase. We find that the precursor-occupied presequence translocase and its associated import motor display compositional dynamics. Regulatory subunits and co-chaperones for mtHsp70 are recruited from a pool of free proteins into the active translocation machinery. Our analyses demonstrate that during precursor translocation a recharging of the translocase with the stimulatory J-protein Pam18 is required to regulate the activity cycle of the import motor. We suggest that a cycle of co-chaperone replenishment at the translocon is the underlying principle for regulation of mtHsp70’s ATPase activity during matrix protein translocation. Import motor activity maintains a TOM/TIM23 intermediate To assess the regulation of the mitochondrial import motor in the context of a translocating polypeptide chain, we accumulated the purified model matrix protein b 2 (167) Δ -dihydrofolate reductase (DHFR) in saturating amounts in mitochondria. Addition of the DHFR substrate analogue methotrexate (MTX) to in vitro import reactions generates a tightly folded DHFR domain incapable of TOM translocation and thus establishes a TOM/TIM23-accumulated precursor that can be detected on blue native polyacrylamide gel electrophoresis (BN-PAGE; Fig. 1b ) [22] . Temperature-sensitive mutants of mitochondrial Hsp70 (Ssc1 in yeast), affected in either ATP-binding and hydrolysis ( ssc1-3 ) [23] or Tim44 interaction ( ssc1-2 ) [24] , displayed defects in matrix protein import and concomitant TOM/TIM23-supercomplex formation when import reactions were performed under non-permissive conditions ( Fig. 1b , lanes 7–12, and Supplementary Fig. 1 ). To assess whether the ATPase activity of mtHsp70 was also required to retain the precursor in the translocases, we first accumulated the matrix-destined precursor under permissive conditions in ssc1-3 mitochondria. Next, we monitored supercomplex stability after mtHsp70 inactivation by a heat shock ( Fig. 1c ). Under these conditions, a substantial amount of the translocation intermediate was lost upon mtHsp70 inactivation, indicating that the activity of the mitochondrial import motor was also required for holding the arrested precursor intermediate in the translocase ( Fig. 1d ). For comparison, we used a temperature-sensitive mutant ( pam18-66 ) of the J-protein Pam18 (refs 13 , 14 , 15 ). Pam18 inactivation after precursor accumulation led to a similar loss of the TOM/TIM23 supercomplex, as observed in the ssc1-3 mutant. Although previous BN-PAGE analyses indicated that mtHsp70/Tim44 were not a stoichiometric constituents of the TOM/TIM23 supercomplex [25] , subsequent analyses showed that all constituents of the import motor are recovered with the TOM/TIM23 supercomplex when mild affinity isolations are employed [13] , [26] , [27] , [28] , [29] , [30] . Accordingly, at the active translocase, ATP hydrolysis by Hsp70, stimulated by its co-chaperone Pam18, was required to sustain the matrix-destined translocation intermediate. To assess whether the observed defects in precursor maintenance were due to an altered organization of the PAM complex at the presequence translocase, we immunoprecipitated TIM23 complexes together with the associated imported motor in the presence and absence of ATP ( Supplementary Fig. 2a ). In the presence of ATP, only mtHsp70 was released from the TIM23 complex to a significant extent ( Supplementary Fig. 2b ). Thus, the nucleotide-bound state of mtHsp70 apparently did not cause dissociation of other motor subunits from the translocase. In agreement, ssc1-3 mitochondria displayed no apparent change in TIM23 or PAM complex organization ( Supplementary Fig. 3a ). In contrast, pam18-66 mitochondria displayed a selective loss of the J-protein Pam18 from the translocase ( Supplementary Fig. 3b , the mutant form of Pam18 displays faster migration in SDS–polyacrylamide gel electrophoresis (SDS–PAGE) analyses and is efficiently recognized by the anti-Pam18 antiserum, lane 1 versus 2). Interestingly, despite the fact that Pam18 and Pam16 are considered to form a stable complex [11] , [16] , [26] , [31] , the inhibitory Pam16 remained translocase-associated in pam18-66 mitochondria. Thus, we concluded that the observed loss of motor function and concomitant instability of the translocation intermediate could be attributed to defective ATPase cycling at the import motor. This malfunction can be accounted for by two distinctly different phenomena: (i) in the ssc1-3 mutant, the enzyme function of mtHsp70 is directly affected, (ii) in the pam18-66 mutant, the ATPase function of mtHsp70 is affected by the selective dissociation of the J-protein Pam18 from the translocase and thus indirectly caused through a lack of co-chaperone activity. Import motor defects affect matrix protein import and translocation of tightly folded domains [23] , [28] . In contrast to mutants of the co-chaperones, pam17 Δ and mgr2 Δ cells are viable, but are characterized by growth retardation [28] , [32] . Nevertheless, pam17 Δ and mgr2 Δ mitochondria displayed selective matrix protein import defects ( Fig. 1e ) [28] , [32] , [33] . In contrast, both mutant mitochondria were capable of motor-independent inner membrane sorting, a process that is driven by the membrane potential across the inner membrane alone ( Fig. 1f and ref. 28 ). Pam17 appears to primarily act during early steps of the matrix transport process [33] . A lack of Pam17 causes a partial dissociation of the Pam16/18 module from the TIM23 complex and concomitantly affects import and motor activity [28] . Mgr2 has only recently been identified as a subunit of the TIM23 complex. The small protein spans the inner membrane twice exposing N- and C-terminus into the intermembrane space. Mgr2 has been found to crosslink to precursors in transit and to promote the association between presequence translocase and respiratory chain complexes [32] . However, the molecular function of Mgr2 in protein transport remains elusive. Interestingly, although Mgr2 is not a motor constituent, mgr2 Δ mitochondria display a selective import defect for matrix-destined precursors ( Fig. 1e,f ) [32] . In contrast to other mutants with matrix-import specific transport defects, the import phenotype manifests itself despite the fact that all PAM components remain associated with the presequence translocase ( Supplementary Fig. 3c ). Although it is intuitive that motor activity and thus matrix import are affected upon loss of co-chaperones or inactivation of individual motor subunits, the fact that matrix import could be compromised in the presence of all PAM constituents at the translocase was surprising and hinted upon an altered arrangement or dynamics. Therefore, we further analysed the inward driving activity of the import motor in mgr2 Δ mutant mitochondria. This assay relies on the fact that in the presence of an inward-driving activity, provided by the mitochondrial import motor, the precursor’s stably folded DHFR domain (in the presence of the inhibitor MTX) is closely ‘pulled’ against the outer membrane and thereby protected from externally added protease [24] . Considering the mutant matrix import defect, we imported an established sorted precursor DHFR-fusion (cytochrome b 2 (1-220)-DHFR) that contained a folded heme-binding domain and determined protease resistance in the presence of MTX [27] , [28] . In mgr2 Δ mitochondria, the stalled polypeptide chain displayed a significant loss of protease resistance ( Fig. 1g,h and Supplementary Fig. 3d ). Similarly, protease sensitivity of the translocation intermediate was observed in the tested pam mutants because of the lack of import-driving activity ( Fig. 1h and Supplementary Fig. 3e ). Thus, we concluded that in the absence as well as in the presence of PAM constituents at the translocase, motor activity could be compromised. Assembly of subunits into TIM23 and PAM complexes Based on our findings, we speculated that proper motor function required the dynamic exchange of subunits at the active TIM23 complex. To address this hypothesis experimentally, we first imported Tim and Pam proteins into Tim23 ProtA -containing mitochondria and analysed if these were capable of incorporating into TIM23/PAM complexes ( Fig. 2a ). The specific co-purification of the Tim and Pam subunits with Tim23 PA was monitored by western blotting ( Fig. 2b ). While matrix-destined substrates of the translocase (Atp2 or Su9-DHFR) were not significantly co-isolated after they were imported ( Fig. 2c,d ), radiolabelled Tim23, Tim50 ( Fig. 2e ), Tim17, Tim21 ( Fig. 2f ) and Mgr2 ( Fig. 2g ) were assembled into the TIM23 complex with different efficiencies ( Fig. 2i ). Moreover, the import motor constituents, Pam16 ( Fig. 2c ), Pam17 ( Fig. 2d ), Pam18 ( Fig. 2e ) and Tim44 ( Fig. 2h ), were assembled into the PAM complex and were thus co-isolated with Tim23 PA ( Fig. 2i ). As only a fraction of Ssc1 is associated with the PAM complex at steady state, assembly of the translocase-associated portion of Ssc1 could not be faithfully monitored ( Fig. 2d ). In summary, although previous studies had only reported assembly of Tim23 and Tim17 into the translocation machinery [25] , [34] , here we show that all Tim and Pam subunits, except Ssc1, could be assembled to the translocase in organello . 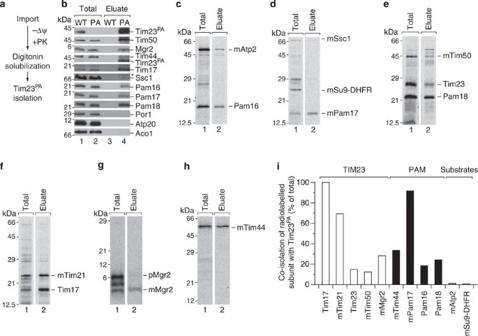Figure 2: Assembly of Tim and Pam components into the translocase. (a) Experimental setup to assay assembly of radiolabelled subunits into the TIM23 translocase. (b) WT and Tim23PAmitochondria were digitonin solubilized and subjected to IgG chromatography. Analysis by SDS–PAGE and western blotting using the indicated antisera. Total: 5%, eluate: 100%. *Eluted IgG. (c–h) Mixtures of radiolabelled import substrates (Atp2 and Su9-DHFR), Tim23 and Pam proteins were imported into Tim23PA-containing mitochondria. Subsequent to proteinase K treatment, Tim23PAwas isolated as described inb. Analysis by SDS–PAGE and digital autoradiography. Total: 5%, eluate: 100%. m, mature; p, precursor. (i) Quantification of autoradiograms shown inc–h. Co-isolation efficiency of radiolabelled proteins with Tim23PAwas normalized to isolation efficiency of [35S]Tim17. Figure 2: Assembly of Tim and Pam components into the translocase. ( a ) Experimental setup to assay assembly of radiolabelled subunits into the TIM23 translocase. ( b ) WT and Tim23 PA mitochondria were digitonin solubilized and subjected to IgG chromatography. Analysis by SDS–PAGE and western blotting using the indicated antisera. Total: 5%, eluate: 100%. *Eluted IgG. ( c – h ) Mixtures of radiolabelled import substrates (Atp2 and Su9-DHFR), Tim23 and Pam proteins were imported into Tim23 PA -containing mitochondria. Subsequent to proteinase K treatment, Tim23 PA was isolated as described in b . Analysis by SDS–PAGE and digital autoradiography. Total: 5%, eluate: 100%. m, mature; p, precursor. ( i ) Quantification of autoradiograms shown in c – h . Co-isolation efficiency of radiolabelled proteins with Tim23 PA was normalized to isolation efficiency of [ 35 S]Tim17. Full size image Import motor subunits integrate into the active translocase Based on this observation, we asked whether the Tim and Pam subunits could also assemble into the active presequence translocase, occupied by a translocating precursor protein. In a first step, the matrix protein b 2 (167) Δ -DHFR was accumulated in sub-saturating amounts, generating the TOM/TIM23 translocation intermediate. Subsequently, radiolabelled proteins of interest were to be imported through the remaining vacant presequence translocases. The stabilized translocation intermediates could then be isolated via tagged TIM23 or TOM complex subunits to analyse integration of imported Tom or Tim proteins, respectively ( Fig. 3a ). To establish the experimental conditions, chemical amounts of a matrix-destined precursor were accumulated in a TOM/TIM23 supercomplex. The blocking efficiency of the translocase was determined through reisolation of mitochondria after precursor accumulation and subsequent import of radiolabelled matrix proteins ( Supplementary Fig. 4a ). Conditions of intermediate translocase saturation were chosen for further experiments and we ascertained that TOM/TIM23 supercomplexes could still be isolated from solubilized mitochondria containing His-tagged Tom22 ( Supplementary Fig. 4b ). 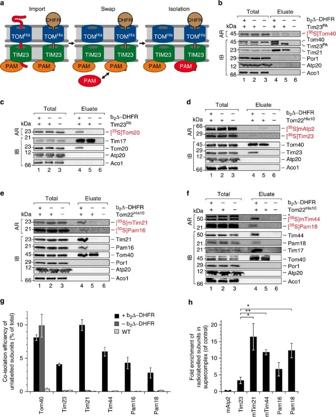Figure 3: Import motor subunits assemble into an active translocase complex. (a) Schematic presentation of recruitment assay of TIM23 and PAM subunits. Approximately half of the import sites in Tom22His10mitochondria were saturated with MTX-treated b2(167)Δ-DHFR. After mitochondria reisolation, radiolabelled proteins were imported. Upon Δψ dissipation, one part was subjected to proteinase K (PK) treatment and the remaining fraction was used to co-isolate the TIM23 complex using the His10 tag on Tom22. (b) Recruitment assay for [35S]Tom40 in Tim23PAmitochondria. After semi-saturating b2(167)Δ-DHFR (b2Δ-DHFR) arrest, radiolabelled Tom40 was imported. Subsequently, the sample was subjected to IgG chromatography. As a control, proteins were imported into WT and Tim23PAmitochondria in the absence of an arrested precursor as indicated. Samples were analysed by SDS–PAGE, digital autoradiogaphy and western blotting. Total: 5%, eluate: 100%. (c) Recruitment assay as described inbfor [35S]Tom20 in Tim23PAmitochondria. Analysis was performed as inb. Total: 5%, eluate: 100%. (d–f) Recruitment assay as described inawas performed with [35S]Tim23 and [35S]Atp2 (d), [35S]Tim21 and [35S]Pam16 (e) or [35S]Tim44 and [35S]Pam18 (f) in Tom22His10mitochondria. A fraction of the sample was PK treated after the import to determine the imported fraction. As a control, the proteins were imported into WT and Tom22His10mitochondria lacking accumulated precursor. Analysis as inb. Total: 5%, eluate: 100%. (g) Quantification of protein (non-labelled) co-isolation with Tom22His10as ind–f. Co-isolation efficiencies are shown as % of imported (PK treated; mean±s.e.m.,n=3). (h) Quantification of co-isolation of radiolabelled subunits with Tom22His10as ind–f. The fold of enrichment (in the presence versus absence of accumulated precursor) of the imported radiolabelled subunits in the Tom22His10isolation is shown (mean±s.e.m.,n=3, **a=0.01, *a=0.05, one-tailedt-test for unequal variances). AR, autoradiogram; IB, immunoblot. Figure 3: Import motor subunits assemble into an active translocase complex. ( a ) Schematic presentation of recruitment assay of TIM23 and PAM subunits. Approximately half of the import sites in Tom22 His10 mitochondria were saturated with MTX-treated b 2 (167) Δ -DHFR. After mitochondria reisolation, radiolabelled proteins were imported. Upon Δψ dissipation, one part was subjected to proteinase K (PK) treatment and the remaining fraction was used to co-isolate the TIM23 complex using the His10 tag on Tom22. ( b ) Recruitment assay for [ 35 S]Tom40 in Tim23 PA mitochondria. After semi-saturating b 2 (167) Δ -DHFR (b 2 Δ-DHFR) arrest, radiolabelled Tom40 was imported. Subsequently, the sample was subjected to IgG chromatography. As a control, proteins were imported into WT and Tim23 PA mitochondria in the absence of an arrested precursor as indicated. Samples were analysed by SDS–PAGE, digital autoradiogaphy and western blotting. Total: 5%, eluate: 100%. ( c ) Recruitment assay as described in b for [ 35 S]Tom20 in Tim23 PA mitochondria. Analysis was performed as in b . Total: 5%, eluate: 100%. ( d – f ) Recruitment assay as described in a was performed with [ 35 S]Tim23 and [ 35 S]Atp2 ( d ), [ 35 S]Tim21 and [ 35 S]Pam16 ( e ) or [ 35 S]Tim44 and [ 35 S]Pam18 ( f ) in Tom22 His10 mitochondria. A fraction of the sample was PK treated after the import to determine the imported fraction. As a control, the proteins were imported into WT and Tom22 His10 mitochondria lacking accumulated precursor. Analysis as in b . Total: 5%, eluate: 100%. ( g ) Quantification of protein (non-labelled) co-isolation with Tom22 His10 as in d – f . Co-isolation efficiencies are shown as % of imported (PK treated; mean±s.e.m., n =3). ( h ) Quantification of co-isolation of radiolabelled subunits with Tom22 His10 as in d – f . The fold of enrichment (in the presence versus absence of accumulated precursor) of the imported radiolabelled subunits in the Tom22 His10 isolation is shown (mean±s.e.m., n =3, ** a =0.01, * a =0.05, one-tailed t -test for unequal variances). AR, autoradiogram; IB, immunoblot. Full size image Using these conditions, we generated the translocation intermediate and afterwards imported radiolabelled [ 35 S]Tom40 ( Fig. 3b ) or the receptor [ 35 S]Tom20 ( Fig. 3c ). Assembly into the translocation intermediate was monitored by isolating the TIM23 complex using protein A-tagged Tim23. Pre-existing Tom40 ( Fig. 3b ) and Tom20 ( Fig. 3c ) co-purified with the TIM23 complex in the presence of an accumulated precursor ( Supplementary Fig. 4c ). In contrast to imported [ 35 S]Tom40, [ 35 S]Tom20 incorporated into the preformed translocation intermediate complex ( Fig. 3b,c and Supplementary Fig. 4d ). To assess TIM23 and PAM recruitment into the TOM/TIM23 supercomplex, we used Tom22 His10 mitochondria for isolation ( Fig. 3a ). Pre-existing Tim23 was only co-purified with TOM in the presence of accumulated precursor ( Fig. 3d,g ). As expected, a radiolabelled matrix-targeted substrate protein of the TIM23 complex ([ 35 S]Atp2) was not co-isolated. Neither did imported [ 35 S]Tim23 incorporate significantly into the translocation intermediate ( Fig. 3d,h ). Thus, the channel-forming subunits of both translocases, Tom40 and Tim23, were unable to assemble once the precursor was accumulated in a two membrane-spanning manner. This finding agreed with BN-PAGE analyses, indicating a lack of Tim23 assembly into an occupied translocase [25] . We next analysed Tim21, Pam16, Tim44 and Pam18 ( Fig. 3e,f ). For all these Tim and Pam subunits, the preexisting proteins were efficiently recovered with the TOM/TIM23 supercomplex ( Fig. 3g ). Similarly, the radiolabelled, imported proteins ([ 35 S]Tim21, [ 35 S]Pam16, [ 35 S]Tim44 and [ 35 S]Pam18) were specifically incorporated into the translocation intermediate. Pam18 recruitment was approximately twice as efficient as integration of the inhibitory Pam16 ( Fig. 3h ). For comparison, we assembled both proteins into the resting presequence translocase and observed a similar ratio ( Supplementary Fig. 4e ). It should be noted that although this assay only allows to analyse the integration of subunits, we assume that a release occurs to a similar extent as indicated by the presence of a free pool of Pam16 and Pam18 in mitochondria [11] , [26] , [30] , [31] , [35] . Thus, our experiments demonstrated that Tim21 and subunits of the PAM complex can be recruited into a precursor-occupied and active translocase, a state that requires import motor activity for formation and maintenance. Mutant mitochondria affect recruitment of Pam18 to TIM23 The observed recruitment of subunits agreed with the hypothesis that subunit exchange at the translocase was required for efficient motor function during precursor transport. Accordingly, matrix import and motor-driving defects could be in principle triggered through inactivation/loss (as in ssc1-3 or pam18-66 ) of motor subunits or stalling of their dynamics at the active translocon and concomitant deregulation of the mtHsp70 cycle. To test this model directly, we analysed the recruitment of the co-chaperones Tim44, Pam16 and Pam18 to the resting TIM23 complex in mutant mitochondria ( Fig. 4a ). Despite the observed matrix translocation defect, mgr2 Δ mitochondria displayed wild-type-like motor association at steady state ( Supplementary Fig. 3c ). Therefore, we utilized the mgr2 Δ mutant to assess co-chaperone dynamics at the translocase. The recruitment of newly imported [ 35 S]Pam18 to the presequence translocase was drastically reduced in the absence of Mgr2 ( Fig. 4b and Supplementary Fig. 4f ). In contrast, association of imported [ 35 S]Pam16 and [ 35 S]Tim44 with the TIM23 complex was not affected in mgr2 Δ mitochondria. As a control, we assessed co-chaperone recruitment in the absence of Tim21. tim21 Δ mitochondria display no matrix import defects [27] , [36] and a motor activity closely resembling the wild-type situation ( Fig. 1h ) [27] . Interestingly, Tim21 and the Pam16/18 J-complex appear to associate with the TIM23 complex in a mutually exclusive manner [27] , [29] , [30] , [32] , [34] . Thus, as expected, in tim21 Δ mitochondria an increased recruitment of newly imported [ 35 S]Pam18 to the translocase was observed compared with wild type ( Fig. 4b and Supplementary Fig. 4f ). Interestingly, although [ 35 S]Pam16 and [ 35 S]Pam18 displayed a differential recruitment to the TIM23 complex in mgr2 Δ mitochondria, in the absence of Tim21, [ 35 S]Pam16 association to the presequence translocase resembled that of [ 35 S]Pam18. In contrast, [ 35 S]Tim44 association to the presequence translocase was wild-type-like in both mutants ( Fig. 4b and Supplementary Fig. 4f ). Accordingly, the selective defect observed for Pam18 recharging at the presequence translocase correlated with the matrix import phenotype of the mgr2 Δ mutant. At the same time, recruitment of the motor subunits Tim44 and Pam16 was not affected. Thus, we conclude that a replenishment of Pam18 at the active translocon is required for the regulation of mtHsp70’s ATPase cycle during the translocation process. Moreover, these analyses suggest that Pam18 and Pam16 can be recruited independent of each other into the import motor. 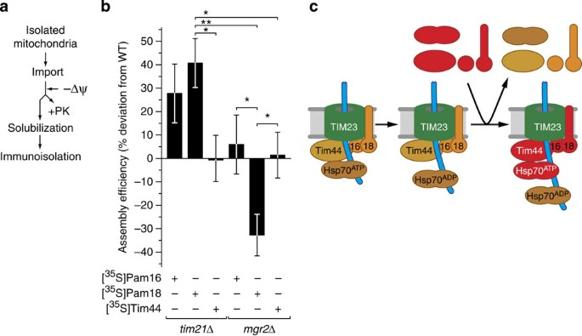Figure 4: Translocase recruitment of motor subunits is affected in mutant mitochondria. (a) Experimental scheme assaying the assembly of radiolabelled subunits to the resting TIM23 translocase. (b) [35S]Pam16, [35S]Pam18 or [35S]Tim44 were imported into isolatedtim21Δ ormgr2Δ and the corresponding WT mitochondria. After Δψ dissipation, an aliquot of the sample was proteinase K treated (imported fraction) or solubilized with digitonin and subjected to α-Tim23 co-immunoprecipitation. Samples were analysed by SDS–PAGE, digital autoradiography and western blotting. The quantification shows the assembly efficiency of the radiolabelled subunits (% of imported, normalized to the unlabelled protein and Tim23) in mutants as % difference to the respective WT control (mean±s.e.m.,n=3, *a=0.05, **a=0.01, one-tailedt-test for unequal variances). (c) During polypeptide translocation TIM23 complex-associated motor subunits are recruited to the import channel. Recharging of the translocase with co-chaperones is required to support continuous precursor translocation. Figure 4: Translocase recruitment of motor subunits is affected in mutant mitochondria. ( a ) Experimental scheme assaying the assembly of radiolabelled subunits to the resting TIM23 translocase. ( b ) [ 35 S]Pam16, [ 35 S]Pam18 or [ 35 S]Tim44 were imported into isolated tim21 Δ or mgr2 Δ and the corresponding WT mitochondria. After Δψ dissipation, an aliquot of the sample was proteinase K treated (imported fraction) or solubilized with digitonin and subjected to α-Tim23 co-immunoprecipitation. Samples were analysed by SDS–PAGE, digital autoradiography and western blotting. The quantification shows the assembly efficiency of the radiolabelled subunits (% of imported, normalized to the unlabelled protein and Tim23) in mutants as % difference to the respective WT control (mean±s.e.m., n =3, * a =0.05, ** a =0.01, one-tailed t -test for unequal variances). ( c ) During polypeptide translocation TIM23 complex-associated motor subunits are recruited to the import channel. Recharging of the translocase with co-chaperones is required to support continuous precursor translocation. Full size image Two major questions on the regulation of the mitochondrial import motor have remained elusive. How is the activity of Hsp70 regulated during the progression of the translocating polypeptide and why is a free pool of the co-chaperones Pam16 and Pam18 present in mitochondria? Our results demonstrate that in the presence of a translocating polypeptide chain, the TOM/TIM23 supercomplex does not form a passive and stable entity to accommodate the polypeptide chain during membrane passage but displays remodelling of its constituents. Subunits of the presequence translocase and its associated import motor are recruited into the translocation intermediate ( Fig. 4c ). The analyses of mutant mitochondria, affected in translocase and motor dynamics, revealed that the sole presence of co-chaperones at the TIM23 complex is insufficient to maintain mtHsp70 in an import competent state. Interestingly, in a mutant that displayed a reduced integration of the J-protein Pam18 into the translocase a specific motor-dependent matrix import defect is observed, probably due to a deregulation in the ATPase cycle of mtHsp70. Hence, we conclude that the observed integration of import motor subunits, especially Pam18, into the precursor-occupied presequence translocase is required for continuous mtHsp70 activity and hence productive precursor progression into the mitochondrial matrix. The association of the membrane-bound co-chaperones with the Tim23 channel unit is a prerequisite for the spatially controlled mtHsp70 regulation in mitochondria [27] , [31] , [37] . However, beside the translocase-associated portion of the co-chaperones Pam16 and Pam18, a significant non-translocase pool of the proteins has been found in mitochondria [11] , [26] , [30] , [31] , [35] . This, situation is now explained by the observed dynamics of the active translocase. A cycle of co-chaperone recruitment and subsequent release would allow coupling of the ATPase cycle of mtHsp70 to the activity of the translocon. At the resting translocase, Pam18 and Pam16 form a complex in which the J-protein is incapable of mtHsp70 activation [12] , [16] , [18] . Our finding that the recruitment of Pam18 into the active translocase is more efficient than that of Pam16 and that in case of the mgr2 Δ mutant both proteins display a different mode of translocase recruitment ( Figs 3h and 4b ) suggests a model in which the J-protein is recruited as a free protein and concomitantly becomes inactivated by associating with Pam16 at the translocase. It is tempting to speculate that precursor-dependent activation of Pam18 at the translocase could subsequently lead to a loss of Pam18 from the translocase. Hence, Pam18 needs to be recharged at the translocase in order to maintain progressive mtHsp70 activity. Thus, we conclude that such a replenishment cycle of the translocase’s co-chaperone Pam18 drives the ATP hydrolysis of the import motor in the precursor-occupied translocase and thus precursor transport along the presequence pathway. Similar to mitochondria, translocases of the endoplasmatic reticulum and chloroplasts use Hsp70-powered import motors that require regulation of their ATPase cycle in the context of the corresponding translocase by membrane-bound co-chaperones. It is tempting to speculate that our findings may represent a general scheme as to how the regulation of translocation-promoting chaperones is coupled to the activity of the import channels. Yeast growth Temperature-sensitive mutants ( tim54-11 (ref. 38 ), pam16-3 (ref. 26 ), pam18-66 (ref. 13 ) and ssc1-3 (ref. 23 )) and their respective wild types were grown in YPG at 24 °C. Deletion mutants were grown at 30 °C in YPG (1% yeast extract, 2% peptone, 3% (w/v) glycerol), mgr2 Δ was shifted for 24 h to 39 °C before harvesting [32] . Mitochondria were prepared as previously described [26] . Import of precursor proteins Precursor proteins were radiolabelled by translation in reticulocyte lysate (Promega) in the presence of [ 35 S]methionine. Import into mitochondria was performed in import buffer (250 mM sucrose, 10 mM MOPS/KOH pH 7.2, 80 mM KCl, 2mM KH 2 PO 4 , 5 mM MgCl 2 , 5 mM methionine and 1% fatty acid-free BSA) at 25 °C in the presence of 2 mM nicotinamide adenine dinucleotide and 2 mM ATP. An ATP regenerating system (5 mM creatine phosphate (CP) and 0.1 mg ml −1 creatine kinase (CK)) was added for imports exceeding 20 min. Temperature-sensitive strains were incubated in energy-free import buffer for 15 °C at 37 °C (heat shock) and subsequently ATP, NADH, CK and CP were added. Unless stated otherwise, the membrane potential was dissipated using 1 μM valinomycin, 8 μM antimycin A and 20 μM oligomycin. Proteinase K (PK) treatment was performed using 40 μg ml −1 for 10 min on ice. PK was inactivated using 4 mM phenylmethylsulphonyl fluoride (PMSF) for 10 min on ice. Samples were washed with SEM buffer (250 mM sucrose, 20 mM MOPS/KOH pH 7.2 and 1 mM EDTA) and further analysed. For import competition experiments, b 2 (167) Δ -DHFR was first imported in the presence of 5 μM MTX for 15 min at 25 °C. Mitochondria were reisolated and resuspended in energized import buffer for import of the radiolabelled precursor. The inward driving activity was tested as previously described [26] . Temperature-sensitive strains were incubated in energy-free import buffer for 15 °C at 37 °C (heat shock) and subsequently ATP, NADH, CK and CP were added. Afterwards, radiolabelled b 2 (220)-DHFR was imported for 15 min at 25 °C in the presence of 5 μM MTX. After dissipation of the membrane potential using 1 μM valinomycin, a sample was taken (Δ t =0 min) and the precursor was chased at 25 °C. Samples were removed after 1, 5 and 10 min and PK treated. Samples were analysed using SDS–PAGE and digital autoradiography. The amount of PK-resistant intermediate was quantified in relation to the generated amount of intermediate (Δ t =0 min). For comparison of different mutants, Δ t was set to 5 min. Maintenance of TOM/TIM23 supercomplex Purified b 2 (167) Δ -DHFR was imported in the presence of 5 μM MTX for 15 min at 25 °C. Temperature-sensitive mutants were optionally subjected to a heat shock. Reactions were chased after addition of 1 μM valinomycin for 30 min at 25 or 37 °C. Then, samples were solubilized for BN-PAGE using 1% digitonin buffer. BN-PAGE was performed according to the standard procedures. The samples were analysed by western blot analysis (α-Tim23), the amount of TOM/TIM23 supercomplex was quantified and the supercomplex retained after the 37 °C (restrictive) chase was set in relation to the amount retained after 25 °C (permissive) chase. Protein complex isolations Co-immunoprecipitations using α-Tim23 serum under conditions lacking or containing ATP were performed as described before [24] . Briefly, mitochondria (1 mg ml −1 ) were solubilized in 30 mM Tris/HCl pH 7.4, 80 mM KCl, 5 mM MgCl 2 , 5% (w/v) glycerol, 1 mM PMSF and 1% digitonin for 30 min on ice. For ATP containing reactions, 2 mM ATP was added. Reactions lacking ATP contained 5 mM EDTA instead. Unless indicated otherwise, α-Tim23 co-immunoprecipitations were performed under –ATP conditions. Soluble material was loaded on Protein A sepharose loaded with α-Tim23 for 1.5 h at 4 °C. Columns were washed with the respective solubilization buffer containing 0.3% digitonin and samples were eluted with 100 mM glycine pH 2.8. In order to address the ability of Pam18, Pam16 and Tim44 to assemble to the TIM23 complex, Tim23 co-immunoprecipitations were performed after import of the radiolabelled proteins. After analysis by digital autoradiography and western blotting, the co-isolation efficiency of the imported radiolabelled proteins was normalized to the co-precipitation efficiency of the unlabelled proteins and to the purification efficiency of the bait Tim23. Isolation of the TOM/TIM23 supercomplex occupied with the arrested substrate b 2 (167) Δ -DHFR was carried out with isolated Tom22 His10 mitochondria. To this end, semi-saturating amounts of MTX-treated b 2 (167) Δ -DHFR were imported for 15 min, the mitochondria were reisolated into energized import buffer and the radiolabelled subunit was imported for 20 min at 25 °C. After dissipation of the membrane potential, one part of the reaction was subjected to PK treatment (omitted for TOM subunits). This was used to determine the import efficiency. The remainder was subjected to a SEM wash and solubilization on ice at 1 μg μl −1 in 30 mM Tris/HCl pH 7.4, 150 mM NaCl, 10% glycerol, 0.1 mM EDTA, 1% digitonin, 30 mM imidazole and 1 mM PMSF for 30 min at 4 °C, the soluble material was loaded on NiNTA-agarose and incubated for 1 h at 4 °C. The beads were washed with solubilization buffer containing 0.2% digitonin and 80 mM imidazole. Samples were eluted with washing buffer containing 200 mM imidazole. Isolation of the TOM/TIM23 supercomplex using Protein A-tagged Tim23 were performed similarly, except that the buffers used contained 20 mM Tris/HCl pH 7.4, 1 mM EDTA and lacked imidazole. The material was bound to IgG-sepharose and eluted using sample buffer. The association of Tim and Pam subunits with Tim23 PA was analysed by importing the radiolabelled subunits for 45 min at 25 °C. After dissipation of the membrane potential and PK treatment (40 μg ml −1 ), the mitochondria were pelleted and washed with SEM buffer. Solubilization was performed at 1 mg ml −1 in 20 mM Tris/HCl pH 7.4, 150 mM NaCl, 10% glycerol, 1 mM EDTA, 1% digitonin and 2 mM PMSF on ice for 30 min. Soluble material was loaded on IgG-sepharose for 2 h at 4 °C. After washing with solubilization buffer containing 0.3% digitonin, samples were eluted with 100 mM glycine pH 2.8, precipitated with 15% trichloroacetic acid and analysed by SDS–PAGE and western blotting. Miscellaneous b 2 (167) Δ -DHFR was purified from E. coli as described before [25] . SDS–PAGE and western blotting were performed by standard procedures. Proteins were detected using enhanced chemiluminescence (GE Healthcare) or fluorescently labelled antibodies (LI-COR). Contrast adjustments were performed using Photoshop CS4 (Adobe). Quantifications were performed using ImageQuant TL (GE Healthcare) using a rolling ball background subtraction. Uncropped scans of the most important western blots and gels can be found in Supplementary Fig. 5. How to cite this article: Schulz, C. et al. Remodelling of the active presequence translocase drives motor-dependent mitochondrial protein translocation. Nat. Commun. 5:4349 doi: 10.1038/ncomms5349 (2014).